Multiple intrinsically identical single-photon emitters in the solid state Emitters of indistinguishable single photons are crucial for the growing field of quantum technologies. To realize scalability and increase the complexity of quantum optics technologies, multiple independent yet identical single-photon emitters are required. However, typical solid-state single-photon sources are inherently dissimilar, necessitating the use of electrical feedback or optical cavities to improve spectral overlap between distinct emitters. Here we demonstrate bright silicon vacancy (SiV − ) centres in low-strain bulk diamond, which show spectral overlap of up to 91% and nearly transform-limited excitation linewidths. This is the first time that distinct single-photon emitters in the solid state have shown intrinsically identical spectral properties. Our results have impact on the application of single-photon sources for quantum optics and cryptography. Single transform-limited photons are an essential resource [1] , [2] , [3] for many quantum interference experiments, as indistinguishability between photons allows path-of-origin information to be erased. This makes it possible to investigate fundamental quantum optics phenomena, which have applications in quantum imaging [4] , quantum computing [1] and quantum repeaters [2] . Interactions between indistinguishable photons from multiple emitters can also be used to create entangled quantum states over macroscopic physical distances [3] . However, to date, it has been proven difficult to achieve indistinguishability between distinct single-photon sources. Individual trapped ions in vacuum are a natural source of identical photons, limited primarily by their independent motion [5] . The solid-state environment overcomes this limitation and allows distinct emitters to be addressed, but also adds complexity and local variations to the emitter environment. It has been necessary to use optical cavities [6] and/or electrical tuning [7] , [8] , [9] to interfere photons from distinct emitters [10] in the solid state. Quantum dots and single molecules have demonstrated transform-limited linewidths over short timescales, allowing interference between photons from the same emitter [6] , [11] and physically separated emitters [7] . Colour centres in diamond, located deep within an ultrapure lattice, show excellent photostability and are attractive single-photon sources. The negative nitrogen vacancy (NV − ) centre is well studied and has been used for early photonics applications [12] , [13] , but its broad spectral emission is ill-suited to single-photon technologies [3] . The negative silicon vacancy (SiV − ) centre in diamond has promising spectral properties [14] , [15] , [16] . It has a strong optical transition with a prominent zero-phonon line (ZPL) at 737 nm and only a weak phonon sideband [17] , [18] , [19] , [20] , [21] . Structurally, it comprises a silicon atom located between adjacent vacancies in the diamond lattice [15] , [22] , [23] ( Fig. 1a ). The strong ZPL has sparked interest, but large variation in spectral properties between individual sites [16] has limited the value of SiV − as a single-photon emitter. Here we obtain highly uniform, narrow linewidths from single SiV − centres in a low-strain bulk diamond. 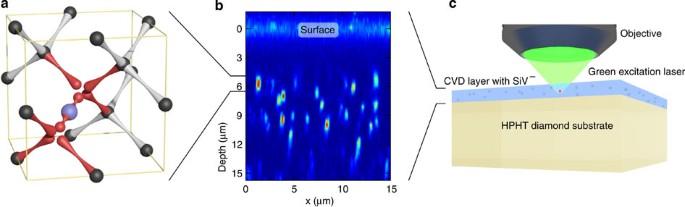Figure 1: Silicon vacancy centres in diamond. (a) Physical structure of the SiV−centre in the diamond lattice, with a silicon atom lying in between adjacent vacancies. (b) Fluorescence confocal image showing the depth profile of single SiV−centres beneath the diamond surface (corrected for refractive index). (c) The SiV−centres were present in a single crystal chemical vapour deposition (CVD) diamond layer, and had been incorporated during growth due to silicon doping of the plasma. The CVD layer was grown homoepitaxially on a low strain, high-pressure high-temperature (HPHT) diamond substrate and investigated from the top. Figure 1: Silicon vacancy centres in diamond. ( a ) Physical structure of the SiV − centre in the diamond lattice, with a silicon atom lying in between adjacent vacancies. ( b ) Fluorescence confocal image showing the depth profile of single SiV − centres beneath the diamond surface (corrected for refractive index). ( c ) The SiV − centres were present in a single crystal chemical vapour deposition (CVD) diamond layer, and had been incorporated during growth due to silicon doping of the plasma. The CVD layer was grown homoepitaxially on a low strain, high-pressure high-temperature (HPHT) diamond substrate and investigated from the top. Full size image Lifetime-limited flourescence linewidth The diamond sample was prepared on a high-pressure high-temperature diamond substrate, as this fabrication technique can produce high crystalline quality with low strain. A layer of ultrapure diamond was overgrown on this ‹001›-oriented substrate with chemical vapour deposition, allowing precise control of impurity concentrations. Silicon was introduced to the plasma and incorporated into the diamond at concentrations below 1 p.p.b. (see Methods). Single SiV − defects formed during growth were observed by fluorescence confocal microscopy ( Fig. 1b,c ). Photon antibunching measurements provided confirmation of single-photon emission. At 4 K, the ZPL consists of four lines as a result of optically allowed transitions between doublet ground and excited states [24] , [25] ( Fig. 2a,b ). Each of these transitions was resonantly excited and fluorescence was detected in the sideband. Scanning the laser frequency produced photoluminescence excitation (PLE) spectra, shown in Fig. 2c for a single emitter. 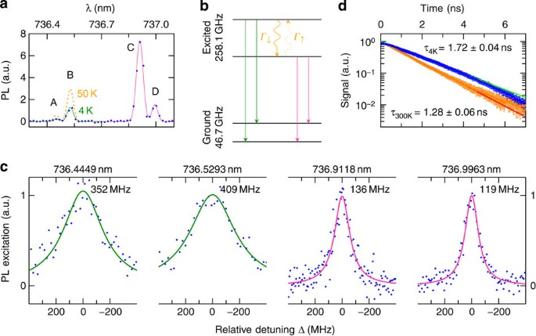Figure 2: Linewidths near the transform limit. (a) The SiV−ZPL has a four-line fine structure (linewidth limited here by spectrometer resolution). The left-hand pair of lines are a mirror image of the right-hand pair, but they have much lower intensity at 4 K. These higher energy lines regain intensity with increasing temperature, and the dotted line illustrates the relative intensity at 50 K. (b) This fine structure arises from transitions between a doublet excited state and a doublet ground state that both have zero-field splittings. Population is exchanged between the two excited state branches, but at low temperature the upward rateΓ↑is slow relative to the state lifetime. The downward exchange rateΓ↓dominates the relaxation within the excited state, which accounts for the loss of emission intensity for the high-energy pair of lines. (c) Excitation spectra of the four lines that comprise the SiV−ZPL (amplitudes normalized). The higher energy lines are wider, consistent with a shorter effective lifetime due to thermalization between the two excited state branches. (d) The radiative decay lifetime of SiV−increases from 1.28 ns at room temperature to 1.72 ns at 4 K, corresponding to a transform-limited PLE linewidth of 94 MHz. The error bars indicate s.d. across 15 randomly selected SiV−centres. Figure 2: Linewidths near the transform limit. ( a ) The SiV − ZPL has a four-line fine structure (linewidth limited here by spectrometer resolution). The left-hand pair of lines are a mirror image of the right-hand pair, but they have much lower intensity at 4 K. These higher energy lines regain intensity with increasing temperature, and the dotted line illustrates the relative intensity at 50 K. ( b ) This fine structure arises from transitions between a doublet excited state and a doublet ground state that both have zero-field splittings. Population is exchanged between the two excited state branches, but at low temperature the upward rate Γ ↑ is slow relative to the state lifetime. The downward exchange rate Γ ↓ dominates the relaxation within the excited state, which accounts for the loss of emission intensity for the high-energy pair of lines. ( c ) Excitation spectra of the four lines that comprise the SiV − ZPL (amplitudes normalized). The higher energy lines are wider, consistent with a shorter effective lifetime due to thermalization between the two excited state branches. ( d ) The radiative decay lifetime of SiV − increases from 1.28 ns at room temperature to 1.72 ns at 4 K, corresponding to a transform-limited PLE linewidth of 94 MHz. The error bars indicate s.d. across 15 randomly selected SiV − centres. Full size image The pair of lines at shorter wavelengths (higher energy), here labelled lines A and B, had full-width at half maximum (FWHM) of 352 and 409 MHz. The pair of lines at longer wavelengths were considerably narrower at 136 MHz (line C) and 119 MHz (line D). All of these PLE spectra were recorded at minimal laser intensities to avoid power broadening. To compare these linewidths with their expected Fourier-transform limit, pulsed 532 nm excitation was used to measure the excited-state lifetime for several individual SiV − centres ( Fig. 2c ). A decay time of 1.72±0.04 ns was measured at 4 K. Our measured result for line D is therefore only 26% over the transform-limited linewidth of 94 MHz. Spectral stability of SiV emitters At 4 K, 71% of the total ZPL flourescence is contained in line C. Combined with the Debye–Waller factor of 70% [26] , this means that half of the total SiV − flourescence is emitted into the almost transform-limited line C. In addition, this transition is known to arise from a single (axial) dipole moment [24] , [25] . These properties are ideal for coupling to narrowband cavities and waveguides, and for single-photon interference experiments, including quantum cryptography. The following discussion therefore focusses on line C. Over a period of 7 h, the line position was recorded for a single SiV − centre ( Fig. 3a ). The variation in line position was found to be ±4 MHz, which is within the 95% confidence interval for this parameter obtained from a Lorentzian fit. The fact that we observe no spectral diffusion highlights the ability of SiV − to produce indistinguishable photons over long periods of time. No blinking was observed for any of the SiV − sites measured in this study. 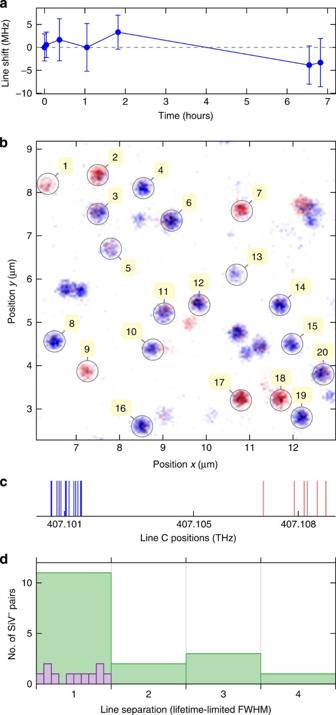Figure 3: Stability and uniformity of single SiV−centres. (a) No measurable spectral diffusion was detected over a period of 7 h. Error bars represent a 95% confidence interval for the line position extracted from a Lorentzian fit. (b) PLE spectra were measured for each of the 20 resolvable single SiV−centres in this confocal image (numbered). The image is a composite of two scans performed at orthogonal excitation polarizations, and so the apparent colour of the sites indicates its orientation in the crystal lattice. (c) Position of line C for each of the 20 SiV−centres. (d) Histogram of the shift between adjacent sites inc. The primary bins are 94 MHz wide corresponding to the transform-limited linewidth, and the composition of the first bin is illustrated in ten sub-bins. Eleven SiV−pairs had separations <94 MHz, and four pairs had separations <30% of the lifetime-limited linewidth. Figure 3: Stability and uniformity of single SiV − centres. ( a ) No measurable spectral diffusion was detected over a period of 7 h. Error bars represent a 95% confidence interval for the line position extracted from a Lorentzian fit. ( b ) PLE spectra were measured for each of the 20 resolvable single SiV − centres in this confocal image (numbered). The image is a composite of two scans performed at orthogonal excitation polarizations, and so the apparent colour of the sites indicates its orientation in the crystal lattice. ( c ) Position of line C for each of the 20 SiV − centres. ( d ) Histogram of the shift between adjacent sites in c . The primary bins are 94 MHz wide corresponding to the transform-limited linewidth, and the composition of the first bin is illustrated in ten sub-bins. Eleven SiV − pairs had separations <94 MHz, and four pairs had separations <30% of the lifetime-limited linewidth. Full size image PLE spectra were recorded for all 20 clearly resolvable SiV − sites in an arbitrary scan region, shown in Fig. 3b . On a {001} surface, the projections of ‹111›-aligned SiV − centres form two orthogonal sets [24] . Scanning with two orthogonal laser polarizations (encoded in colour) revealed the set to which each site in the region belonged [24] . The line position for each site is illustrated in Fig. 3c . Within each orientation set the sites are closely spaced, although the distinct orientations are separated by about 5 GHz. Figure 3d shows a histogram of the shifts between consecutive sites. Out of the 20 centres, 11 pairs of SiV − have separations <1 transform-limited FWHM. This means that for a randomly chosen site there is >50% probability of finding a second site in this scan region whose line is displaced by <1 FWHM. The two closest sites had lines separated by only 6 MHz (within the confidence interval of the fit), meaning a spectral overlap of at least 91%. Notably, this spectral overlap was achieved without external tuning of the spectral position. SiV incorporation in solid immersion lens An advantage to solid-state emitters over trapped ions is their reliable addressing, which allows direct incorporation into photonic and plasmonic devices. SiV − ensembles have been coupled into cavities [27] , and here we incorporate single SiV − centres into a solid-immersion lens (SILs) to demonstrate their readiness for applications ( Fig. 4a ). SILs allow increased collection of flourescence from high refractive index materials [28] , [29] , which is particularly useful during cryogenic experiments. Well-coupled SiV − centres were identified by scanning the depth profile with a confocal microscope. The SIL enhanced flourescence collection by about a factor of ten, giving a saturation flourescence up to I sat =730 kc s −1 . Using an oil-immersion objective on a flat surface, SiV − produced I sat =200 kc s −1 , which is comparable to a single NV − centre or bright molecule under the same conditions ( Fig. 4b ). 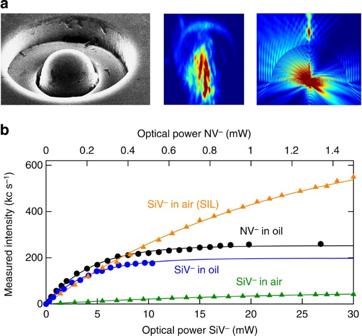Figure 4: SiV−incorporation into a SIL. (a) Scanning electron microscope image of a single SIL fabricated in the diamond surface. The vertical cross-section confocal image (centre) shows an intensity profile in the SIL with enhanced fluorescence detection for SiV−centres near the focus. This is in qualitative agreement with the simulated emission intensity (right) for a single dipole located at the centre of the solid immersion lens (calculated with finite-difference time-domain numerical package). (b) Using an air objective (numerical aperture (NA)=0.95), the saturation count rateIsatfor SiV−under a SIL (730 kc s−1) is enhanced by more than a factor of 10 compared with an equivalent single SiV−under a planar surface nearby (Isat=56 kc s−1). To more easily compare SiV−with other emitters, a high performance (NA=1.35) oil-immersion objective was used at room temperature. SiV−sites showIsat=200 kc s−1, which is comparable to single NV−centres (Isat=252 kc s−1). Figure 4: SiV − incorporation into a SIL. ( a ) Scanning electron microscope image of a single SIL fabricated in the diamond surface. The vertical cross-section confocal image (centre) shows an intensity profile in the SIL with enhanced fluorescence detection for SiV − centres near the focus. This is in qualitative agreement with the simulated emission intensity (right) for a single dipole located at the centre of the solid immersion lens (calculated with finite-difference time-domain numerical package). ( b ) Using an air objective (numerical aperture (NA)=0.95), the saturation count rate I sat for SiV − under a SIL (730 kc s −1 ) is enhanced by more than a factor of 10 compared with an equivalent single SiV − under a planar surface nearby ( I sat =56 kc s −1 ). To more easily compare SiV − with other emitters, a high performance (NA=1.35) oil-immersion objective was used at room temperature. SiV − sites show I sat =200 kc s −1 , which is comparable to single NV − centres ( I sat =252 kc s −1 ). Full size image Although narrow spectral lines were measured for the lower-energy transitions, the higher energy pair of lines were broader by nearly a factor of three. It is important to account for this extra width of lines A and B, and further information is provided by photoluminescence measured with a spectrometer. At 4 K, lines C and D are much brighter than the higher-energy lines ( Fig. 2a ), which correspond to transitions from the upper branch of the excited state ( Fig. 2b ). With increasing temperature, the high-energy lines gain relative intensity, indicating that thermal relaxation occurs in the SiV − excited state. The downward exchange rate Γ ↓ adds to the rate of decay to the ground state and reduces the effective lifetime of the upper branch. Consequently, lines A and B are broadened and lose intensity in photoluminescence. The upward exchange rate depends on the Boltzmann factor, making it small but still measurable at 4 K. This additional rate out of the lower branch accounts for half of the exta linewidth above the transform limit for lines C and D. To explain the observed homogeneity between distinct centres, we reconsider the energy level scheme in Fig. 2b . The ground and excited states have E symmetry [15] , [24] , [25] and are split due to spin–orbit interaction [24] . In general, strain and electric fields can perturb these states to result in line shifts and increased splittings. Electric fields may be produced by nearby charged impurities and, therefore, vary across small spatial scales. The precise correspondence between orientation and line position for each SiV − measured here suggests that strain, which can be nearly uniform over a 7 × 7-μm region, is more influential than electric fields. The large spin–orbit splittings of 46.7 GHz (258.1 GHz) in the ground (excited) state help to make SiV − unresponsive to small transverse strains. This occurs because the effect of such strain is a small perturbation until strain splitting increases to about the magnitude of spin–orbit. We observed this effect in the ground-state splitting measured between lines C and D, which varied much less (±1 GHz) than line position across the 20 sites and showed no correlation with orientation. This implies that the observed line shift results from axial strain. The inversion symmetry of SiV − (refs 15 , 24 ) reduces the influence of small axial strain, as inverting the strain direction does not change line shift. Our observations indicate that this shielding has a lower threshold than provided by spin–orbit for transverse strain. Despite the presence of residual strain in this sample region we were still able to find identical emitters. The spectral properties we have presented establish SiV − as an attractive single-photon emitter. For such applications, it is usually of interest to have a high quantum yield, meaning that the probability of photon emission is high for each excitation event. Measuring the absolute quantum yield is difficult, because it is not possible to collect all of the photons emitted by a colour centre. Here we have reported saturation fluorescence, but the presence of poorly understood metastable states [30] prevents a deduction of absolute quantum yield for SiV − from these data. It seems, however, that SiV − has a lower quantum yield than NV − , which has similar saturation flourescence but a longer excited-state lifetime of 13 ns [12] . We found the SiV − decay lifetime to be shorter (1.28±0.06 ns) at room temperature than at 4 K ( Fig. 2d ). This is consistent with a thermally activated non-radiative decay path [17] , [26] , [31] and indicates an improvement of the SiV − quantum yield at low temperature. It may be possible to disable this non-radiative decay path and dramatically improve the quantum yield. This could explain how SiV − centres in nanodiamonds grown on iridium were able to produce flourescence rates up to 6.2 Mc s −1 (ref. 32 ). Another nuance in interpreting saturation flourescence is that photons are measured across the entire emission band of a colour centre (including the phonon sideband). For sources of indistinguishable single photons, the absolute quantum yield is less important than the ‘effective’ yield of photons in the desired transform-limited spectral line. The strong ZPL of SiV − gives it a significant advantage in this respect, and here we have established that line C can contain up to 50% of the total flourescence. Our results show that a single SiV − centre can provide indistinguishable photons at a collectable rate on the order of hundreds of kc s −1 . In summary, we have demonstrated a uniform single-photon source in the solid state without requiring external tuning of the optical properties. We observe nearly transform-limited linewidths, without spectral diffusion, which would allow high spectral overlap between single photons emitted from distinct sources. The production of multiple, independent single-photon emitters with identical properties is essential to the scalability of a number of schemes that use entangled photons, including quantum computing with linear optics, and is expected to form a fundamental resource in quantum optics technologies. The SiV − centre is therefore promising for such applications. Sample preparation A ‹001›-oriented plate cut from a low-strain, type-IIa, high-pressure high-temperature crystal (Sumitomo Electric Industries, Ltd) was used as a substrate for microwave plasma chemical vapour deposition. High-purity H 2 and CH 4 source gas, specified to 99.999% 12 C isotopic enrichment (Cambridge Isotope Laboratories CLM-392) was used to produce the plasma. The residual N 2 concentration was <0.1 p.p.b. for H 2 and <1 p.p.b. for CH 4 . The total gas pressure, microwave power, methane concentration ratio (CH 4 /H 2 ), growth duration and substrate temperature employed were 120 Torr, 1.4 kW, 4%, 24 h and 950–1,000 °C, respectively. The homoepitaxial layer thickness estimated from the weight difference between initial substrate and after the growth was ~60 μm giving a growth rate of 2.4 μm h −1 . Cathodoluminescence spectra (15 kV acceleration voltage, 2 × 10 −7 A incident beam current) taken at room temperature in a wavelength range from 200 to 800 nm provided information on the crystalline quality and optically active impurities. Emission from free-exciton recombination was observed from most of the growth surface, in addition to a weak signal at 738 nm, which is assigned to SiV − . The reaction vessel of microwave plasma chemical vapour deposition contains mainly stainless steel and molybdenum. Quartz glass (SiO 2 ) was used for the windows of the vessel. When homoepitaxial film was grown under low microwave power, no SiV − fluorescence was observed. Increasing the microwave input power caused the plasma to extend and etch material from the quartz, picking up silicon. In this study, a 6H-SiC single-crystal plate was also used as a silicon source to allow increased doping of grown diamond. The SiC plate was inserted between the diamond substrate and a molybdenum sample holder. It was possible to incorporate SiV − during growth at concentrations below 0.2 μm 3 (~1 × 10 −3 p.p.b.). Incorporation of silicon occurred relatively uniformly over the whole lateral direction. Optical measurements The sample was mounted in a continuous flow helium cryostat capable of cooling to 4 K. Single SiV − centres were imaged using a home-built confocal microscope. The excitation laser beam (532 nm) was focused onto the diamond surface through a 0.95-numerical aperture microscope objective (or 1.35 numerical aperture oil-immersion objective for room temperature measurements). The objective was scanned to produce confocal images of sample regions. Fluorescence was collected by the same objective, filtered with a 725- to 775-nm band-pass filter and focused through a 25-μm pinhole before detection on an avalanche photodiode. After the pinhole, the flourescence could also be sent to a spectrometer to acquire spectra from single sites. Using a high-resolution grating (1,596 grooves per mm) allowed the 4-four component fine structure to be resolved. PLE measurements were performed on the same setup, but using a Titanium:Sapphire laser with 50 kHz linewidth for excitation. This laser could scan across the entire ZPL and detection was performed on the sideband by switching the filter to a 750- to 810-nm band-pass. Decay lifetime of the excited state was measured by changing the excitation laser to a Titanium:Sapphire pumped optical parametric oscillator, producing 50 fs pulses at 80 MHz repetition rate. This optical parametric oscillator was set to 532 nm to excite SiV − off-resonantly. The avalanche photodiode signal was analysed using a PicoQuant TimeHarp counting card, with a resolution of 29 ps. SIL fabrication SILs were produced in a region of the sample known to contain a medium density of SiV − centres at a depth of 2.5–6 μm below the surface. The site density was high enough to assure a reasonable probability of coupling a SIL to a colour centre. The fabrication process was performed with a Helios Nanolab 600 Focused Ion Beam lithography system. Each SIL had a radius of 7 μm and a depth of 7 μm. The SIL images were taken with a Helios Nanolab 600 Focused Ion Beam lithography system. How to cite this article: Rogers, L. J. et al. Multiple intrinsically identical single-photon emitters in the solid state. Nat. Commun. 5:4739 doi: 10.1038/ncomms5739 (2014).